An engineered dimeric protein pore that spans adjacent lipid bilayers The bottom-up construction of artificial tissues is an underexplored area of synthetic biology. An important challenge is communication between constituent compartments of the engineered tissue, and between the engineered tissue and additional compartments, including extracellular fluids, further engineered tissue and living cells. Here we present a dimeric transmembrane pore that can span two adjacent lipid bilayers, and thereby allow aqueous compartments to communicate. Two heptameric staphylococcal α-hemolysin pores were covalently linked in an aligned cap-to-cap orientation. The structure of the dimer, (α7) 2 , was confirmed by biochemical analysis, transmission electron microscopy and single-channel electrical recording. We show that one of two β-barrels of (α7) 2 can insert into the lipid bilayer of a small unilamellar vesicle, while the other spans a planar lipid bilayer. The (α7) 2 pores spanning two bilayers were also observed by transmission electron microscopy. A major challenge in synthetic biology is the construction of tissue-like materials. Lipid vesicles have been used as minimal cells (or protocells) [1] , [2] , [3] , [4] , but far less work has been done on minimal tissues, that is, assemblies of small aqueous compartments with tissue-like properties [5] . We have suggested that aqueous droplets connected through droplet interface bilayers [6] might be used to build functional compartmented assemblies, and significant progress has been made in this area [7] , [8] , [9] . An important functional criterion of a minimal cell or tissue is communication with the external environment. Further, in a minimal tissue, the compartments must be able to communicate with each other. To that end, the staphylococcal α-hemolysin (αHL) pore has been used to mediate the transfer of small molecules across the bilayers of lipid vesicles [10] . The αHL pore can also allow compartments in droplet networks to communicate chemically and electrically with each other, and allow the entire assembly to communicate with the external environment [8] . These examples require individual bilayers to be spanned by protein pores, but it would also be advantageous to be able to connect vesicles or compartmented networks of vesicles through their encapsulating bilayers. Previously described methods, such as the drawing of membranous nanotubes to connect vesicles, require external micromanipulation techniques [11] . In favourable circumstances, a simpler and self-assembling alternative would be to use a protein that spans two bilayers ( Fig. 1a ), the issue addressed in the present work. Double bilayers are a recurrent feature in nature and occur in organelles, such as mitochondria, chloroplasts and other plastids, autophagosomes and cell nuclei. Both small and large molecules are ferried across the double membranes of organelles by using transiently interacting proteins spanning each of the bilayers, for example, the TIM/TOM complex of mitochondria [12] , or through permanently associated protein complexes spanning the two bilayers, for example, the nuclear pore complex [13] . A notable example of a protein that spans two bilayers is the gap junction, where the interdigitating extracellular loops of hemichannels or connexons in individual bilayers are connected by a network of hydrogen bonds and salt bridges to form full channels [14] , [15] , [16] . 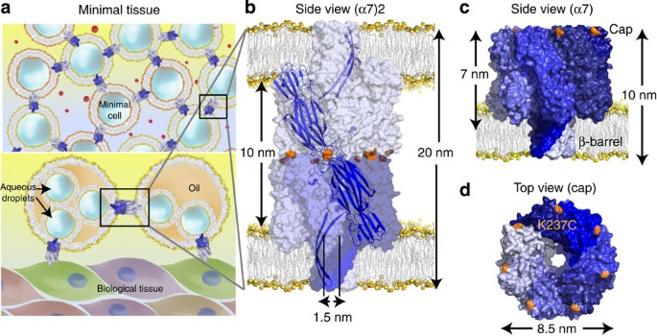Figure 1: An engineered αHL pore dimer. (a) Minimal tissue models. Upper panel: minimal cells communicating through protein conduits that span both bilayers. Lower panel: monolayer-encased droplet networks8interconnected and linked to biological tissues through protein conduits. (b) Space-filling model of the engineered pore dimer, (α7)2, in which two α7 units (the normal form of the αHL pore) are linked cap-to-cap and can span two bilayers simultaneously. (c) The α7 units were covalently attached through disulphide bonds between cysteine residues (orange) at position 237 in the αHL K237C mutant. The cysteine residues are located on the cap of the α7 heptamer, one on each subunit. (d) Top view of the cap and the location of the cysteine residue at position 237 (orange) in α7. The space-filling models of α7 (PDB 7AHL) and (α7)2were created in PyMOL. Figure 1: An engineered αHL pore dimer. ( a ) Minimal tissue models. Upper panel: minimal cells communicating through protein conduits that span both bilayers. Lower panel: monolayer-encased droplet networks [8] interconnected and linked to biological tissues through protein conduits. ( b ) Space-filling model of the engineered pore dimer, (α7) 2 , in which two α7 units (the normal form of the αHL pore) are linked cap-to-cap and can span two bilayers simultaneously. ( c ) The α7 units were covalently attached through disulphide bonds between cysteine residues (orange) at position 237 in the αHL K237C mutant. The cysteine residues are located on the cap of the α7 heptamer, one on each subunit. ( d ) Top view of the cap and the location of the cysteine residue at position 237 (orange) in α7. The space-filling models of α7 (PDB 7AHL) and (α7) 2 were created in PyMOL. Full size image Inspired by the structure of gap junctions, we have engineered a dimeric αHL pore, (α7) 2 , in which two αHL heptamers (α7) are covalently linked by disulphide bonds. (α7) 2 formed spontaneously during the purification of an αHL cysteine mutant that had been designed to allow cap-to-cap coupling. The two β-barrels of the construct are able to insert simultaneously into two different bilayers and, hence, form a conduit between two aqueous compartments ( Fig. 1b ). Disulphide-bonded tubules have previously been obtained from the hexameric ring of Pseudomonas aeruginosa Hcp1 ( [17] ) and from the undecameric ring of Bacillus stereothermophilus Trp RNA-binding attenuation protein [18] , but neither of these structures interact with lipid bilayers. Design of the (α7) 2 pore Our inspiration for (α7) 2 was the hexameric connexon protein, which forms gap junctions between two adjacent biological cells [14] , [15] , [16] . The flat cap of the heptameric αHL pore (α7) [19] offered the possibility of connecting two α7 units cap-to-cap, to yield a dimer with the bilayer-spanning β-barrels pointing away from each other ( Fig. 1b ). To covalently link the two α7 units, a surface-exposed cap residue, Lys-237, was mutated to cysteine ( Fig. 1c ). The K237C mutation has been studied previously and has no effect on the hemolytic activity of monomeric αHL towards rabbit erythrocytes, which requires heptamer formation, even when the cysteine is modified with a bulky chemical group [20] ( Supplementary Fig. S1a ). The unitary conductance of the heptameric (α7) K237C pore in planar lipid bilayers was 857±6 pS (mean±s.e.m; n= 169, N= 9, where n is number of individual events in N independent experiments) in 1 M KCl, 25 mM Tris HCl and 50 μM EDTA, pH 8, which is similar to the value for wild-type (WT) α7 ( [21] ). Molecular dynamics simulations of (α7) 2 The structural viability of a cap-to-cap (α7) 2 dimer of the K237C mutant was evaluated by molecular dynamics (MD) simulations. Two α7 units were docked cap-to-cap in PyMOL, and disulphides were formed between cysteine–thiol pairs in GROMACS [22] . (α7) 2 was solvated in a buffer containing 500 mM NaCl, and a 1 ns all-atom MD simulation was performed. In the energy-minimized structure of (α7) 2 , the seven disulphides did not provoke steric clashes between the other interface residues ( Supplementary Fig. S2a ). Energy analysis revealed favourable overall electrostatic interactions and Lennard–Jones potential energy between the α7 caps ( Supplementary Fig. S2b ). (α7) 2 forms spontaneously during K237C purification A D8H6 peptide tag was placed at the carboxy terminus of the αHL K237C monomer (α1; M app ~33,200) to aid purification by immobilized metal affinity chromatography (Ni-NTA agarose). After separation of K237C/D8H6 from the Escherichia coli cell lysate, a mixture of α1, monomer dimer (α1) 2 , α7 and a species of M app ~190,000 was obtained. We anticipated that the latter was (α7) 2 . The D8H6 tag on the C terminus of αHL promotes premature oligomerization of WT α1 into α7 (Stephen Cheley, unpublished results). Therefore, we believe that α1 spontaneously oligomerizes to α7, which subsequently forms (α7) 2 during purification. α7 is known to be stable in the sample buffer used for SDS–polyacrylamide gel electrophoresis [23] . The spontaneously oligomerized K237C α7 carried seven D8H6 tags and, hence, considerably more negative charge compared with WT α7. The reduced hydrodynamic radius of the folded α7 structure in SDS and the additional negative charges per heptamer caused α7 to migrate quickly during SDS–polyacrylamide gel electrophoresis [24] , with M app ~120,000 rather than M app ~230,000, based on its molecular mass. The dimer, (α7) 2 , too would be expected to migrate more quickly than anticipated, based on its mass, and therefore we attributed the M app ~190,000 band, lying above the α7 band, to (α7) 2 . Structural characterization of (α7) 2 To confirm that the M app ~190,000 species in SDS–polyacrylamide gels ( Fig. 2a ) was (α7) 2 , formed of α7 units linked through disulphide bonds, we extracted the band from a gel in 10 mM Tris HCl and 1 mM EDTA, pH 8, and treated the protein with 3 M βME for 15 min at 25 °C, which yielded α7 only (lane 4, Fig. 2b ). Upon heating the M app ~190,000 species at 95 °C for 10 min in the absence of a reducing agent, it dissociated into two species, which were identified as α1 and (α1) 2 (lane 3, Fig. 2b ). The relative intensities of the α1 and (α1) 2 bands were 18 and 17 absorbance units, respectively. Therefore, (α7) 2 ( M app ~190,000) is composed of α1 and (α1) 2 in a ratio of 2:1 (mol/mol). When (α7) 2 ( M app ~190,000) was treated with 3 M βME for 15 min at 25 °C, followed by heating in 3 M βME at 95 °C for 10 min, only α1 was formed (lane 5, Fig. 2b and Supplementary Fig. S1b ). These experiments showed that the cysteines introduced into the cap domain had been oxidized to form disulphide bonds, and thereby convert α7 to (α7) 2 . 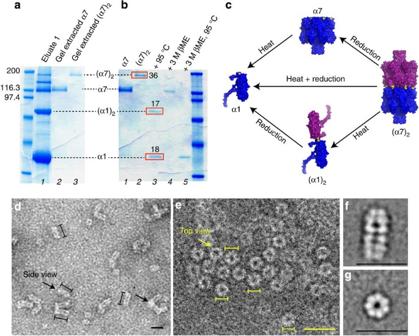Figure 2: Expression, purification and structural characterization of (α7)2. (a) SDS–polyacrylamide gel showing the purification of (α7)2. The Ni2+-NTA-purified αHL mutant K237C/D8H6 contained a mixture of the monomer α1, the monomer dimer (α1)2, the heptamer α7 and the heptamer dimer (α7)2. α7 and (α7)2were purified (lanes 2 and 3) by extraction from a preparative gel (Supplementary Methods). (b) Heating (α7)2at 95 °C for 10 min yielded α1 and (α1)2(red boxes, lane 3) with relative band intensities of 18 and 17 absorbance units, derived from 36 absorbance units of (α7)2(red box, lane 2). To determine whether (α7)2was composed of α7 units linked by disulphide bonds, a sample was treated with 3 M βME for 15 min at 25 °C, which indeed produced α7 (lane 4). Upon heating at 95 °C, followed by reduction with 3 M βME for 15 min at 25 °C, (α7)2dissociated into α1 (lane 5). (c) A model for the structural composition and dissociation of (α7)2based on the electrophoresis studies. (d) Electron micrographs after uranyl acetate staining showing side views (left arrow) of (α7)2as elongated particles of length 19.6±0.2 nm (mean±s.e.m.,n=268) and width 8.4±0.1 nm (mean±s.e.m.;n=96), which correspond to the length (~20 nm) and width (~8.5 nm) of (α7)2derived from a molecular model (Fig. 1b). (α7)2particles were also observed aggregated longitudinally in clusters of three to four molecules, most probably through the hydrophobic β-barrel domains (right arrow). (e) Electron micrographs showing ring views of (α7)2. The average diameter of the particles is 7.8±0.1 nm (mean±s.e.m.,n=131). Lines drawn next to single particles (d: black;e: yellow) denote the boundaries used to measure lengths. (f) Class average of 309 single particles showing the side view. (g) Class average of 224 single particles showing the ring view. (d–g) Scale bars, 20 nm. Figure 2: Expression, purification and structural characterization of (α7) 2 . ( a ) SDS–polyacrylamide gel showing the purification of (α7) 2 . The Ni 2+ -NTA-purified αHL mutant K237C/D8H6 contained a mixture of the monomer α1, the monomer dimer (α1) 2 , the heptamer α7 and the heptamer dimer (α7) 2 . α7 and (α7) 2 were purified (lanes 2 and 3) by extraction from a preparative gel ( Supplementary Methods ). ( b ) Heating (α7) 2 at 95 °C for 10 min yielded α1 and (α1) 2 (red boxes, lane 3) with relative band intensities of 18 and 17 absorbance units, derived from 36 absorbance units of (α7) 2 (red box, lane 2). To determine whether (α7) 2 was composed of α7 units linked by disulphide bonds, a sample was treated with 3 M βME for 15 min at 25 °C, which indeed produced α7 (lane 4). Upon heating at 95 °C, followed by reduction with 3 M βME for 15 min at 25 °C, (α7) 2 dissociated into α1 (lane 5). ( c ) A model for the structural composition and dissociation of (α7) 2 based on the electrophoresis studies. ( d ) Electron micrographs after uranyl acetate staining showing side views (left arrow) of (α7) 2 as elongated particles of length 19.6±0.2 nm (mean±s.e.m., n= 268) and width 8.4±0.1 nm (mean±s.e.m. ; n= 96), which correspond to the length (~20 nm) and width (~8.5 nm) of (α7) 2 derived from a molecular model ( Fig. 1b ). (α7) 2 particles were also observed aggregated longitudinally in clusters of three to four molecules, most probably through the hydrophobic β-barrel domains (right arrow). ( e ) Electron micrographs showing ring views of (α7) 2 . The average diameter of the particles is 7.8±0.1 nm (mean±s.e.m., n= 131). Lines drawn next to single particles ( d : black; e : yellow) denote the boundaries used to measure lengths. ( f ) Class average of 309 single particles showing the side view. ( g ) Class average of 224 single particles showing the ring view. ( d – g ) Scale bars, 20 nm. Full size image (α7) 2 might be formed from structures other than a precisely aligned cap-to-cap structure ( Fig. 1b ), because of the different possible cross-linking patterns between the α7 units ( Supplementary Fig. S3 and Supplementary Note S1 ). However, when the α7 units are linked at three or more positions, that is, by three or more disulphide bonds, only the aligned structure of (α7) 2 is possible ( Supplementary Fig. S3e ). From the ratio of the band intensities of α1 and (α1) 2 in heat-dissociated (α7) 2 ( Fig. 2b ), we deduced that on average ~3.3 out of the 7 cysteines in each α7 unit were oxidized to form disulphide linkages, and hence the majority of the (α7) 2 were aligned along a central axis ( Fig. 1b ). The cap-to-cap structure of (α7) 2 was further investigated by examination of (α7) 2 and α7 by transmission electron microscopy (TEM). α7 was observed only as ring-shaped particles of diameter 8.1±0.1 nm (mean±s.e.m. ; n= 52; data not shown), in accord with previous reports [19] , [25] , [26] . In contrast, both side views and rings were observed in the case of (α7) 2 in a roughly 2:1 ratio ( n= 399, N =4; Fig. 2d ). The (α7) 2 rings looked similar to those of α7 with an average diameter 7.8±0.1 nm (mean±s.e.m. ; n= 131; Fig. 2g and Supplementary Fig. S4 ). Offset (α7) 2 structures ( Supplementary Fig. S3a–d ) could not be discerned among the aligned cap-to-cap structures in the images of the rings ( Fig. 1b and Supplementary Fig. S3e ). The side views of (α7) 2 revealed elongated particles with an average length of 19.6±0.2 nm (mean±s.e.m. ; n= 268) and an average width of 8.4±0.1 nm (mean±s.e.m. ; n= 96; Fig. 2d ), in agreement with the predicted dimensions of a cap-to-cap dimer ( Fig. 1b ). (α7) 2 is a correctly folded structure Proteinase K cleaves at the glycine-rich central domain and near the amino terminus of α1 ( [27] ), regions inaccessible in the α7 structure [28] . α7 extracted from an SDS gel was treated with proteinase K (0.5 mg ml −1 ) and subsequently heated at 95 °C for 10 min, yielding untruncated α1, confirming the previous findings (lanes 5 and 6, Supplementary Fig. S5 ). (α7) 2 treated in the same way, yielded intact α1 and (α1) 2 , and was reduced to intact α7 on treatment with 3 M βME for 15 min at 25 °C (lanes 1–4, Supplementary Fig. S5 ). Therefore, (α7) 2 , similar to α7, has a compact folded structure. Conductance of (α7) 2 suggests it is a longer pore than α7 TEM showed that (α7) 2 inserted into the bilayers of 1-palmitoyl-2-oleoyl-sn-glycero-3-phosphocholine (POPC) liposomes when mixed in a lipid to protein ratio of 100:1 (w/w) ( Fig. 3a ). The average length of (α7) 2 molecules protruding out of single liposomes was 17.0±0.4 nm (mean±s.e.m. ; n= 131), close to the value of 15 nm expected from the molecular model ( Fig. 1b ). As evidenced by electrical recordings, (α7) 2 readily inserted into planar lipid bilayers ( Fig. 3b ). We surmise that one of the α7 β-barrels (which we call the trans -α7 half of the structure) penetrates the bilayer, whereas the other α7 unit ( cis -α7) is surrounded by buffer and perhaps stabilized by residual traces of SDS ( Fig. 3b ). Histograms of the unitary pore currents ( I o ) of (α7) 2 at each of three potentials, +50, +100 and +160 mV, showed at least two populations (red and green, Fig. 3c and Supplementary Fig. S6 ), suggesting the existence of more than one (α7) 2 structure. A double Gaussian function was used to fit the I o histogram of (α7) 2 . At +50 mV, 75% of the (α7) 2 pores had a mean I o of 27±4pA (mean±s.d. ; n =284, N= 18; 1 M KCl, 25 mM Tris HCl and 50 μM EDTA, pH 8; Fig. 3d , red peak), which is ~64% of the I o value of α7 of 42±4 pA (mean±s.d. ; n= 169, N= 9). The mean I o of the remaining 25% of the (α7) 2 pores was 42±4 pA, (mean±s.d. ; n= 93, N= 18; Fig. 3d , green peak), which corresponds to the value for α7. Therefore, the α7 units in the latter (α7) 2 structures may be offset ( Supplementary Fig. S3a–c and Supplementary Note S1 ). The lower conductance of 75% of the (α7) 2 pores (±4%: ±95% confidence interval, see Supplementary Methods and Fig. 3d , red peak) is consistent with a pore that is longer than α7 ( Supplementary Fig. S3d,e ) and most likely reflects a precisely aligned cap-to-cap orientation. As the probability of insertion of the aligned and misaligned (α7) 2 structures ( Supplementary Fig. S3 ) into the planar lipid bilayer must be similar based on their similar structures, the conductance distribution implies that the major species present is the aligned (α7) 2 structure. 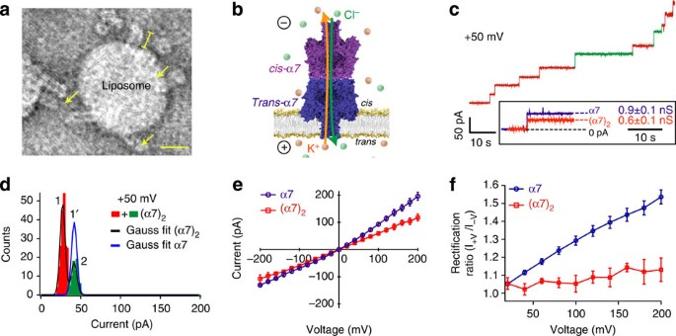Figure 3: Electrical characteristics of (α7)2. (a) TEM view showing (α7)2inserted into the bilayer of a liposome and seen as 17.0±0.4 nm (mean±s.e.m.;n=131) protrusions (yellow) from the liposome surface. Scale bar, 20 nm. (b) (α7)2was electrically characterized in planar lipid bilayers. A bilayer with an area of 1.2 × 104to 3 × 104μm2(determined by capacitance measurements) was formed on an aperture that separated two compartments, both of which contained 1 M KCl, 25 mM Tris HCl and 50 μM EDTA, pH 8 (40). (c) A representative trace showing rapid insertion of (α7)2into a bilayer of DPhPC at +50 mV. Inset: the mean conductance (G) of the majority of the (α7)2pores (red steps) was 570±4 pS (mean±s.e.m.;n=284,N=18). By comparison, α7 gaveG=857±6 pS (mean±s.e.m.;n=169,N=9) under the same conditions. Some (α7)2pores with unitary conductance values similar to α7 were also observed (green steps). (d) Histogram of the open pore currents (Io) of (α7)2at +50 mV showing the two populations (red and green). The meanIovalue of the major (red) peak was 27±4 pA (mean±s.d.;n=284,N=18). In comparison, the meanIoof the minor (green) peak was 42±4 pA (mean±s.d.);n=93,N=18), which is similar to the meanIovalue for α7, 42±4 pA (mean±s.d.;n=169,N=9, blue Gaussian fit). The population of (α7)2pores with the higher meanIovalue (green) is likely to comprise ‘offset’ structures (Supplementary Fig. S3a–c). The pores with the lower meanIovalue (red peak), 27±4 pA can be assigned to structures with precisely aligned cap domains (Fig. 1b). (e) I–V plot for (α7)2(red) compared with that of α7 (blue;N≥3). For the I–V plot of (α7)2, pores withIovalues in the range of 27±4 pA were used. (f) Rectification ratios (I+V/I−V) of α7 and (α7)2were calculated as a function of applied potential. Figure 3: Electrical characteristics of (α7) 2 . ( a ) TEM view showing (α7) 2 inserted into the bilayer of a liposome and seen as 17.0±0.4 nm (mean±s.e.m. ; n =131) protrusions (yellow) from the liposome surface. Scale bar, 20 nm. ( b ) (α7) 2 was electrically characterized in planar lipid bilayers. A bilayer with an area of 1.2 × 10 4 to 3 × 10 4 μm 2 (determined by capacitance measurements) was formed on an aperture that separated two compartments, both of which contained 1 M KCl, 25 mM Tris HCl and 50 μM EDTA, pH 8 ( [40] ). ( c ) A representative trace showing rapid insertion of (α7) 2 into a bilayer of DPhPC at +50 mV. Inset: the mean conductance ( G ) of the majority of the (α7) 2 pores (red steps) was 570±4 pS (mean±s.e.m. ; n= 284, N =18). By comparison, α7 gave G= 857±6 pS (mean±s.e.m. ; n= 169, N =9) under the same conditions. Some (α7) 2 pores with unitary conductance values similar to α7 were also observed (green steps). ( d ) Histogram of the open pore currents ( I o ) of (α7) 2 at +50 mV showing the two populations (red and green). The mean I o value of the major (red) peak was 27±4 pA (mean±s.d. ; n= 284, N= 18). In comparison, the mean I o of the minor (green) peak was 42±4 pA (mean±s.d. ); n= 93, N= 18), which is similar to the mean I o value for α7, 42±4 pA (mean±s.d. ; n= 169, N= 9, blue Gaussian fit). The population of (α7) 2 pores with the higher mean I o value (green) is likely to comprise ‘offset’ structures ( Supplementary Fig. S3a–c ). The pores with the lower mean I o value (red peak), 27±4 pA can be assigned to structures with precisely aligned cap domains ( Fig. 1b ). ( e ) I–V plot for (α7) 2 (red) compared with that of α7 (blue; N≥ 3). For the I–V plot of (α7) 2 , pores with I o values in the range of 27±4 pA were used. ( f ) Rectification ratios ( I +V / I −V ) of α7 and (α7) 2 were calculated as a function of applied potential. Full size image The I–V characteristics of the (α7) 2 and α7 pores differed ( Fig. 3e ). The rectification ratios diverged most strikingly at high potentials. For example, ( I +100 / I −100 ) was 1.29±0.02 (mean±s.e.m. ; N= 5) for α7 and 1.05±0.05 (mean±s.e.m. ; N= 8) for (α7) 2 . Indeed, the I–V characteristics for (α7) 2 were roughly ohmic from negative- to positive-applied potentials, which is consistent with a symmetrical pore structure ( Fig. 3e ). Cyclodextrin binding to (α7) 2 confirms presence of two β-barrels The functional and the structural characteristics of (α7) 2 were further investigated by determining the binding kinetics of the α7 pore adapter, γ-cyclodextrin (γCD) [29] . Large CDs, such as γCD, become lodged near residue N139 in the α7 β-barrel for hundreds of milliseconds, which can be detected electrically as characteristic current blockades [30] . As reported previously, γCD bound to α7 from the trans side of the bilayer only and produced a blockade of 66±1% of I o (percent block±s.e.m. ; n =17,354, N =6) at +50 mV ( Fig. 4a–d ). Under the same conditions, γCD blocked (α7) 2 from both the trans and the cis sides of the bilayer ( Fig. 4e–h ). Blocking from the trans side was observed with 100% success ( n= 33, N= 15, where n is number of pores in N experiments), and from the cis side in 50 out of 56 pores examined (89±8%; percentage of pores blocked±95% confidence interval; n= 56, N= 19; Fig. 4e–h ). Hence, (α7) 2 contains two γCD-binding sites, one facing each side of the bilayer, which is consistent with the presence of two symmetrically placed β-barrels. 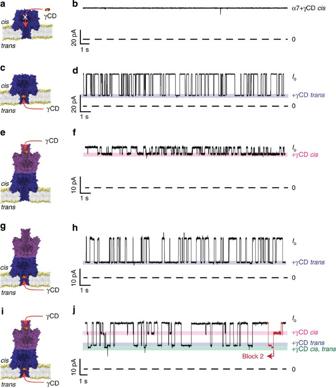Figure 4: γCD binding to α7 and (α7)2. (a,b) When γCD was added to theciscompartment, no blockades of α7 were observed. (c) γCD from thetranscompartment bound within the α7 barrel and produced transient blockades. (d) Representative current trace showing a 66% blockade ofIoupontrans-γCD binding to α7 at +50 mV. (e) γCD bound to (α7)2from theciscompartment. (f) Representative current trace showing a 15% blockade ofIouponcis-γCD binding to (α7)2at +50 mV. (g) γCD also bound to (α7)2from thetranscompartment. (h) Representative current trace showing a 55% blockade ofIoupontrans-γCD binding to (α7)2at +50 mV. (i,j) 40 μM γCD was added to both thecisandtranssides of (α7)2simultaneously. In this case, three blockade levels were observed, which are attributed as follows: (i)cis-only block, 15%; (ii)trans-only block, 55%; (iii) simultaneouscisandtransblock, 61% block (n=4,183, 3,737 and 1,121, respectively andN=6;ndenotes number of individual events inNindependent experiments). The simultaneouscis-andtrans-γCD block was always preceded and followed by acis-only or atrans-only block (for example, see red part of trace:trans→cis+trans→cis). In all traces, the blue and pink bars show thetrans-andcis-γCD blocks, respectively. To investigate γCD binding to (α7)2, only the pores with a unitary conductance of 27±4 pA were used (Fig. 3d, red peak). The current traces were recorded at +50 mV in 1 M KCl, 25 mM Tris HCl and 50 μM EDTA, pH 8, with 80 μM γCD in thecisand/ortranscompartment(s). Figure 4: γCD binding to α7 and (α7) 2 . ( a , b ) When γCD was added to the cis compartment, no blockades of α7 were observed. ( c ) γCD from the trans compartment bound within the α7 barrel and produced transient blockades. ( d ) Representative current trace showing a 66% blockade of I o upon trans -γCD binding to α7 at +50 mV. ( e ) γCD bound to (α7) 2 from the cis compartment. ( f ) Representative current trace showing a 15% blockade of I o upon cis -γCD binding to (α7) 2 at +50 mV. ( g ) γCD also bound to (α7) 2 from the trans compartment. ( h ) Representative current trace showing a 55% blockade of I o upon trans -γCD binding to (α7) 2 at +50 mV. ( i , j ) 40 μM γCD was added to both the cis and trans sides of (α7) 2 simultaneously. In this case, three blockade levels were observed, which are attributed as follows: (i) cis -only block, 15%; (ii) trans- only block, 55%; (iii) simultaneous cis and trans block, 61% block ( n= 4,183, 3,737 and 1,121, respectively and N =6; n denotes number of individual events in N independent experiments). The simultaneous cis- and trans -γCD block was always preceded and followed by a cis -only or a trans -only block (for example, see red part of trace: trans → cis + trans → cis ). In all traces, the blue and pink bars show the trans- and cis- γCD blocks, respectively. To investigate γCD binding to (α7) 2 , only the pores with a unitary conductance of 27±4 pA were used ( Fig. 3d , red peak). The current traces were recorded at +50 mV in 1 M KCl, 25 mM Tris HCl and 50 μM EDTA, pH 8, with 80 μM γCD in the cis and/or trans compartment(s). Full size image γCD, when added to the cis side of a bilayer containing (α7) 2 ( cis -γCD binding), produced a smaller block of I o than trans -γCD binding ( Table 1 ). For example, at +50 mV, cis -γCD gave a 15±1% blockade of I o (percentage block±s.e.m., n =22,344, N =12; where n is the total number of events in N experiments) as compared with 55±2% ( n =11,068, N =7) for trans -γCD binding. The association rate constants ( k on ) were similar for cis- and trans -γCD binding ( Table 1 ). However, the dissociation rate constants ( k off ) for cis -γCD were approximately twice the values determined for trans -γCD binding ( Table 1 ). The physical origins of a smaller block of I o and the slightly weaker cis -γCD binding compared with trans -γCD binding with (α7) 2 might be attributed, respectively, to a leak in the structure ( Supplementary Fig. S3e and Supplementary Note S1 ) and a less compact structure of the cis -α7 β-barrel in (α7) 2 , owing to the absence of a lipid bilayer. Table 1 Kinetic and equilibrium dissociation constants for the interaction of γCD with ( α 7) 2 and α 7. Full size table When γCD was added to both the cis and the trans sides of the bilayer, events were observed that could be attributed to binding to either the cis -α7 unit or the trans -α7 unit, or to both sites at the same time, for example, at +50 mV, simultaneous block, 61±1%; cis block 15±2%; trans block, 57±1% (percentage block of I o ±s.e.m. ; n =1,121, 4,183 and 3,737, respectively, N =6). The simultaneous block was preceded by and followed by either a cis or a trans block ( Fig. 4i ). Phosphate binding confirms aligned structure of M113R (α7) 2 We also examined phosphate anion (P i ), a cis (cap side) blocker of certain α7 mutants [31] . At +20 mV, P i blocked the α7 pore formed from M113R, when added to the cis compartment ( Fig. 5a–c ). The α7 pore remained open when P i was added to the trans compartment (data not shown). We hypothesized that a precise cap-to-cap (α7) 2 , made from the barrel mutant M113R/K237C/D8H6 (MR), would not show P i blockades, as there would be no available entrance for P i ions ( Fig. 5d ). Forty-eight of 65 MR (α7) 2 pores, that is, 74±11% (percentage of pores examined ±95% confidence interval), were not blocked by P i added from the cis side. The population (74%) of (α7) 2 structures obtained from MR with aligned caps, as deduced from P i blocking experiments, corresponded well with the value of 75±4% determined by conductance measurements on K237C pores ( n =377, N= 18; Fig. 3d ). These results in conjunction with the γCD binding, and TEM experiments suggest that a majority of (α7) 2 pores have an aligned cap-to-cap structure. 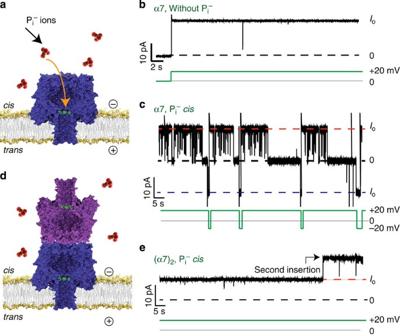Figure 5: Phosphate binding to M113R (α7)2. (a) Phosphate anions (Pi, red) bind and block the heptameric pore (α7) made from MR subunits from thecisside only. (b) MR α7 in the absence of Pi. (c) Representative current trace of a MR α7 pore with Piin theciscompartment. Transient blockades, seen as spikes, and longer blockades are observed at +20 mV. The longer blockades are reversed at −20 mV. (d) Cartoon of the cap-to-cap structure of (α7)2showing that access to the site of blockade in on thetrans-α7 unit is hindered. (e) A representative trace of two (α7)2pores in the presence of Piin theciscompartment. Neither pore bound Piat +20 mV. Inb–e, the broken lines represent theIolevels at +20 mV (red) and −20 mV (blue), and the blocked level (black, 0 pA). The green lines show the applied potential. Partsaanddare not drawn to scale. The experiments were performed in 1 M KCl, 25 mM Tris HCl and 50 μM EDTA, pH 8, with 10 mM sodium phosphate, pH 8 as noted. Figure 5: Phosphate binding to M113R (α7) 2 . ( a ) Phosphate anions (P i , red) bind and block the heptameric pore (α7) made from MR subunits from the cis side only. ( b ) MR α7 in the absence of P i . ( c ) Representative current trace of a MR α7 pore with P i in the cis compartment. Transient blockades, seen as spikes, and longer blockades are observed at +20 mV. The longer blockades are reversed at −20 mV. ( d ) Cartoon of the cap-to-cap structure of (α7) 2 showing that access to the site of blockade in on the trans -α7 unit is hindered. ( e ) A representative trace of two (α7) 2 pores in the presence of P i in the cis compartment. Neither pore bound P i at +20 mV. In b – e , the broken lines represent the I o levels at +20 mV (red) and −20 mV (blue), and the blocked level (black, 0 pA). The green lines show the applied potential. Parts a and d are not drawn to scale. The experiments were performed in 1 M KCl, 25 mM Tris HCl and 50 μM EDTA, pH 8, with 10 mM sodium phosphate, pH 8 as noted. Full size image Of the 65 MR (α7) 2 pores examined, 17 were blocked by P i in a similar manner to MR α7 ( Supplementary Fig. S7 ). Twelve of these 17 MR (α7) 2 pores, that is, 71±22% (percentage of pores examined ±95% confidence interval) had unitary conductance values similar to MR α7. These pores may have had cis -α7 units that were misaligned or misfolded in such a way that P i ions could enter into the trans -α7 unit from the cis compartment. Indeed, when we examined MR (α7) 2 samples that had been freeze-thawed three times, we found that the mean I o was increased by 2 pA and that P i blocking occurred with 14 out of 25 pores ( Supplementary Fig. S8 and Supplementary Note S2 ). (α7) 2 inserts into two lipid bilayers simultaneously The insertion of (α7) 2 into bilayers was examined by TEM. (α7) 2 was mixed with unilamellar L -α-phosphatidylcholine (95%) (egg-PC) liposomes or 10 mol% 1-palmitoyl-2-oleoyl-sn-glycero-3-phospho-(1′– rac- glycerol) (POPG):POPC liposomes in a lipid to protein ratio of 100:1 and 20:1 (w/w), respectively. To prevent the aggregation of liposomes, POPG was added to POPC to make liposomes with a net negative charge. The insertion of one end of (α7) 2 into individual liposomes ( Fig. 3a ) and the simultaneous insertion of both ends into each of two liposomes were observed ( Fig. 6a ). The average length of (α7) 2 structures spanning two liposomes was 12.3±0.7 nm (mean±s.e.m. ; n= 15), close to the value of 10 nm expected from the molecular model ( Fig. 1b ). 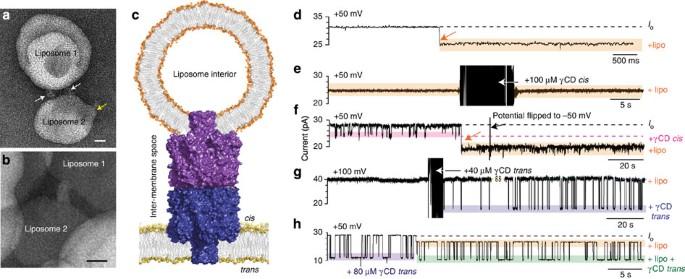Figure 6: Simultaneous insertion of (α7)2into two adjacent lipid bilayers. (a,b) TEM images of (α7)2inserted into two liposomes simultaneously. (α7)2was mixed with (a) 10 mol% POPG:POPC liposomes or (b) egg-PC liposomes in lipid to protein ratios of 20:1 (w/w) and 100:1 (w/w), respectively. Arrows denote (α7)2particles inserted into two liposomes simultaneously (white) and a single liposome (yellow). (c) Insertion into two bilayers was observed in single-channel electrical recordings. Cartoon (not to scale) showing (α7)2with itscis-α7 barrel inserted into a unilamellar liposome and thetrans-α7 barrel inserted into a planar lipid bilayer. (d–h) Representative electrical traces of liposome insertion or liposome-inserted (α7)2pores. (d) Insertion of thecis-α7 barrel of (α7)2into a unilamellar liposome is observed as an irreversible block ofIoof 23±1% (percentage block ofIo±s.e.m.;N=12) at +50 mV. (e) An (α7)2pore that had inserted into a liposome did not display anycis-γCD (100 μM) binding events at +50 mV. (f) Cis-γCD blockades cease after insertion into a liposome at +50 mV. The liposome block could not be reversed by flipping the potential to −50 mV. (g) Upon the addition of γCD (40 μM) to thetransside of an (α7)2pore that had inserted into a liposome, transient binding events (purple box) were detected (+100 mV). (h) If γCD was present on thetransside of (α7)2before liposome insertion,trans-γCD binding events (purple box) continued (green box) after liposome insertion at +50 mV. The experiments were performed in 1 M KCl, 25 mM Tris HCl and 50 μM EDTA, pH 8, with γCD (cisortrans; concentration as noted) and/or liposomes (2.5 mg ml−1,cis), as noted. Figure 6: Simultaneous insertion of (α7) 2 into two adjacent lipid bilayers. ( a , b ) TEM images of (α7) 2 inserted into two liposomes simultaneously. (α7) 2 was mixed with ( a ) 10 mol% POPG:POPC liposomes or ( b ) egg-PC liposomes in lipid to protein ratios of 20:1 (w/w) and 100:1 (w/w), respectively. Arrows denote (α7) 2 particles inserted into two liposomes simultaneously (white) and a single liposome (yellow). ( c ) Insertion into two bilayers was observed in single-channel electrical recordings. Cartoon (not to scale) showing (α7) 2 with its cis -α7 barrel inserted into a unilamellar liposome and the trans -α7 barrel inserted into a planar lipid bilayer. ( d – h ) Representative electrical traces of liposome insertion or liposome-inserted (α7) 2 pores. ( d ) Insertion of the cis -α7 barrel of (α7) 2 into a unilamellar liposome is observed as an irreversible block of I o of 23±1% (percentage block of I o ±s.e.m. ; N= 12) at +50 mV. ( e ) An (α7) 2 pore that had inserted into a liposome did not display any cis -γCD (100 μM) binding events at +50 mV. ( f ) C is -γCD blockades cease after insertion into a liposome at +50 mV. The liposome block could not be reversed by flipping the potential to −50 mV. ( g ) Upon the addition of γCD (40 μM) to the trans side of an (α7) 2 pore that had inserted into a liposome, transient binding events (purple box) were detected (+100 mV). ( h ) If γCD was present on the trans side of (α7) 2 before liposome insertion, trans- γCD binding events (purple box) continued (green box) after liposome insertion at +50 mV. The experiments were performed in 1 M KCl, 25 mM Tris HCl and 50 μM EDTA, pH 8, with γCD ( cis or trans ; concentration as noted) and/or liposomes (2.5 mg ml −1 , cis ), as noted. Full size image To investigate simultaneous insertion into two bilayers by electrical recording, we determined whether the exposed cis β-barrel of (α7) 2 in a planar lipid bilayer could insert into a liposome. First, we found that pre-incubation with unilamellar liposomes (25 mg ml −1 DPhPC (diphytanoyl phosphatidylcholine), 1 M KCl, 25 mM Tris HCl and 50 μM EDTA, pH 8; filter cut-off value, 100 nm diameter) decreased the rate of insertion of (α7) 2 (50 μg ml −1 ) into planar lipid bilayers by >100-fold, presumably because both β-barrels of (α7) 2 had inserted irreversibly into the liposomes. Next, with (α7) 2 already inserted into a planar lipid bilayer, liposomes were added to the cis compartment and a permanent current blockade of 23±1% (percentage of I o ±s.e.m. ; N= 12) was observed at +50 mV in 12 out of 14 experiments ( Fig. 6c ). After being blocked by a liposome, (α7) 2 had a lower unitary conductance over a wide range of applied potentials: −200 to +200 mV ( Supplementary Fig. S9a ), while its rectification properties were little changed ( Supplementary Fig. S9b ). For example, at 100 mV, the rectification ratio ( I +100 / I −100 ) of an (α7) 2 pore inserted into a liposome was 0.96±0.03 (mean±s.e.m., N =3) as compared with 1.05±0.05 (mean±s.e.m., N= 8) for (α7) 2 in the absence of liposomes. The residual current might be explained by one of two scenarios: either by assuming that the attached liposome is porous, because it is penetrated by additional (α7) 2 pores, or by a leak current within the (α7) 2 pore in the planar bilayer ( Supplementary Fig. S10 ). However, the number of (α7) 2 protein molecules present was much smaller than the number of liposomes in the cis compartment, which argues against the first possibility. Further, the consistent magnitude of current blockades caused by liposome insertion favours the second scenario ( Supplementary Note S3 ). cis -γCD blockades cease after liposome insertion To confirm that the observed blockade of (α7) 2 arose because of cis -α7 barrel insertion into a liposome, γCD was added to the cis compartment before and after (α7) 2 liposome insertion. When γCD was added after insertion of (α7) 2 into a liposome, γCD-binding events were not observed ( N =6), confirming that the cis -α7 barrel entrance was inaccessible ( Fig. 6e ). If γCD was already present in the cis compartment before the addition of liposomes, the blocking events ceased upon insertion of the cis -α7 unit into a liposome ( N =4, Fig. 6f ). By contrast, if γCD was present on the trans side before the addition of liposomes, γCD blockades continued even after the insertion of the cis -α7 unit into a liposome ( Fig. 6g ). However, the magnitude of current blockades arising from trans -γCD binding changed from 60±1% (mean±s.e.m.) before insertion to 56±1% after insertion ( n =4,144, N= 5; Supplementary Note S3 ). Therefore, the cis -α7 unit could insert into a liposome, which then occluded the barrel entrance, but produced no effect on the binding properties of the trans -α7 unit, which spanned the planar lipid bilayer. Electrical model of (α7) 2 explains its observed properties To explain the electrical properties of (α7) 2 and the current blockades observed with γCD and liposomes, an electrical model of the pore was constructed ( Supplementary Note S3 ). The model assumes that the cis -α7 and trans -α7 units are resistors, represented by R c and R t , respectively (Supplementary Fig. S11a,b). The values of R c and R t were set to experimentally determined values of the unitary resistance of α7 at −50 mV and +50 mV, respectively. The value for R c was taken at −50 mV, because the orientation of the cis -α7 unit is the opposite of that of trans- α7, and the opposite of that in our usual sign convention. In any event, both values are 1.2 GΩ, because rectification of α7 is weak at low potentials ( Fig. 3e ). Therefore, the resistance of (α7) 2 should be 2.4 GΩ. However, the experimentally determined resistance of the cap-to-cap (α7) 2 pores ( R d ) was 1.8 GΩ, which implies that a leak in the structure of (α7) 2 contributes to the measured conduction through the (α7) 2 pore. The leak could be due to a flow of ions in between the cis -α7 and trans -α7 units or through aqueous channels within the α1 subunits ( Supplementary Fig. S3e ). To account for the leak current, an additional resistor ( R L ) was placed in parallel to R c . By using the experimentally determined values of R d =1.8 GΩ, R c =1.2 GΩ and R t =1.2 GΩ, R L was calculated to be 1.2 GΩ at +50 mV. Current blockades by γCD can be explained with the same electrical model by including an additional resistance R CD . A switch is included to contend with transient binding, that is, the pore with γCD bound has the switch open, whereas the unoccupied pore has the switch closed ( Supplementary Fig. S11c–f ). The overall resistances of the model circuits were calculated ( Supplementary Note S3 ). At +50 mV, the blockades in I o due to cis- and trans -γCD binding are 14% and 56%, respectively ( Supplementary Fig. S11d,e and Supplementary Table S1 ), which match the experimental values of 15±1% and 55±2%, respectively ( Table 1 ). Similarly, the calculated current blockade for simultaneous binding of γCD to both the cis and trans sites is 59% ( Supplementary Fig. S11f ), which is similar to the experimental value of 61±1% at +50 mV. The value of the current block expected upon liposome insertion at +50 mV is computed to be 25% ( Supplementary Fig. S12a ), which agrees well with the experimental liposome blockade of 23±1%. The trans -γCD blockade when the cis -α7 unit is inserted into a liposome is 49% ( Supplementary Fig. S12b ) according to the model, which is reasonably close to the experimental value of 56±1%. Theoretical values of R L and cis- and trans -γCD blocking were calculated by using equations (S3)–(S9) ( Supplementary Note S3 ) at +100 and −50 mV. The predicted values ( Supplementary Table S1 ) correlate well with the experimentally observed values ( Table 1 ). These correlations imply that the calculated value of R L is correct at all the potentials examined. Comparing the values of R L and R c , we infer that the leak amounts to 50%, and to 60%, of the total current going into the trans -α7 unit at +50 mV and −50 mV, and at +100 mV, respectively. We have used protein engineering to build a dimeric pore (α7) 2 that, in a similar way as eukaryotic gap junctions, can span two lipid bilayers to form a conductive pathway. The structure of (α7) 2 was characterized by biochemical assays, TEM and single-channel electrical recordings. The majority of the (α7) 2 comprise two α7 heptamers linked cap-to-cap in a fully aligned fashion through cysteine residues at position 237 ( Fig. 1b–d ). We confirmed the double β-barrel structure of (α7) 2 by investigating the interactions of γCD, which bound to the two β-barrels of (α7) 2 independently. Single-channel electrical measurements showed that the β-barrels of a (α7) 2 pore could span simultaneously a planar lipid bilayer and the bilayer of a small unilamellar lipid vesicle. The bridging of two lipid vesicles by (α7) 2 was also observed by electron microscopy. This paper describes the best attempt so far at the rational design and characterization of a pore that is able to connect two adjacent lipid bilayers. Despite the leak at the cap interface, we believe that the (α7) 2 pore is useful in its present form, for example, for electrical communication across minimal tissues. Further, as the defect has been fully characterized, it should be possible to remedy it in future work. For example, additional disulphide bonds and electrostatic interactions might pull the heptamers closer together, or a covalently attached polymer skirt at the cap interface might reduce ion flow. Extensive studies have shown that the heptameric αHL pore can be engineered to produce a versatile assortment of functionalized pores, with altered properties, including size selection, rectification, triggered activity, reversible gating and blocker binding [7] , [29] , [31] , [32] , [33] . If such properties were introduced into (α7) 2 , the dimeric pore might be used in a variety of contexts. For example, minimal cells endowed with a light-activated (α7) 2 might be used to inject doses of therapeutic or cytotoxic agents directly into living cells [34] , [35] . Minimal cells connected through (α7) 2 might be used to form minimal tissues, that is, collections of communicating compartments ( Fig. 1a , upper panel). A different form of minimal tissue formed of networks of aqueous droplets connected by single lipid bilayers has been under development in our laboratory [6] , [7] , [8] , [9] . Recently, it has been demonstrated that these networks can be encapsulated in small oil drops so that they are separated from the external environment through single bilayers [8] . These encapsulated aqueous droplet networks might be connected to each other through bridges such as (α7) 2 to form extended tissue-like networks ( Fig. 1a , lower panel). As in the case of gap junctions [36] , thousands of (α7) 2 pores might be required to transfer substantial amounts of small molecules across the protocells in minimal tissues. As the αHL pore is capable of spanning the plasma membranes of mammalian cells [34] , it also follows that (α7) 2 might be used to integrate minimal tissues with living cells and tissues by permitting chemical and electrical communication between them, and thereby open up further frontiers in tissue engineering ( Fig. 1a , lower panel). Computational modelling of (α7) 2 Two α7 subunits with the K237C mutation were docked in a cap-to-cap orientation in PyMOL (Schrodinger) such that the cysteines of each α7 aligned with the other. The topology file was generated using GROMACS version 4.0 ( www.gromacs.org ) and was edited to introduce position restraints on the cysteine–thiol atoms. The distance between sulphur atoms adjacent cysteines was fixed at 0.2 nm, which is the S–S bond length. An all-atom MD simulation was performed on the docked structure for 1 ns in 500 mM NaCl buffer using the OPLS-AA/L all-atom force field. The integration time step was 2 fs with an all-bonds constraint. The Particle-Mesh Ewald method [37] was used to compute long-range electrostatic interactions, and the short-range electrostatic cut-off was kept at 1 nm with a Fourier spacing of 0.32. Steric clashes were visualized by using a PyMOL script (show_bumps.py, Thomas Holder) with a van der Waals radius cut-off value of 0.3 Å. Expression and purification of (α7) 2 and the mutant M113R The K237C mutation was introduced into a gene encoding αHL with a D8H6 tag at the C terminus, contained within a pT7 vector [38] , by mutagenic PCR followed by homologous recombination in XL10-Gold ultracompetent E. coli cells (Agilent). The sequences of the primers used in the forward and reverse PCR mutagenesis reactions were 5′-CTATGGATAGATGCGCATCCAAACAACAAACAAATATAG-3′ (forward primer) and 5′-CAGAAGTGGTCCTGCAACTTTAT-3′ (reverse primer, and 5′-CTATATTTGTTTGTTGTTTGGATGCGCATCTATCCATAG-3′ (reverse primer) and 5′-ATAAAGTTGCAGGACCACTTCTG-3′ (forward primer), respectively. Rosetta (DE3) pLysS competent cells (Novagen) were used for protein expression. The αHL proteins α1, (α1) 2 , α7 and (α7) 2 were observed in the cell lysate and purified by Ni 2+ -NTA chromatography. α7 and (α7) 2 were further purified by extraction from SDS–polyacrylamide gels ( Supplementary Methods ). Proteinase K assay Proteinase K (5 mg ml −1 ) was added to purified (α7) 2 (1:9 v/v), and incubated for 5 min at 25 °C, when phenylmethylsulfonyl fluoride was added to a final concentration of 2 mM to inhibit the protease. The samples were analysed by using 10% w/v Bis-Tris SDS–PAGE (Bio-Rad). Single-channel electrical recording All electrical recordings were done by using planar lipid bilayers formed from DPhPC (Avanti Polar Lipids) across a 125-μm aperture in a 30-μm-thick Teflon film with 1 M KCl, 25 mM Tris HCl and 50 μM EDTA, pH 8, as the electrolyte. The αHL proteins were added to the electrically grounded compartment, termed ‘ cis ’ ( Fig. 3b ). Ag/AgCl electrodes were used to apply a bias potential, given as V trans − V cis . The electrical current was amplified with a patch-clamp amplifier (Axopatch 200B, Axon Instruments) and was acquired with a 1 kHz filter at a sampling frequency of 10 kHz. The electrical recordings were post-filtered with low-pass 100 Hz Bessel filter. Experiments reported in the paper were performed with proteins aliquots that had not been freeze-thawed more than once. All chemicals were purchased from Sigma, unless specified otherwise. Phosphate (P i ) binding experiments Stocks of sodium dihydrogen phosphate (NaH 2 PO 4 ; 0.5 M) and disodium hydrogen phosphate (Na 2 HPO 4 ; 0.5 M) were mixed to prepare 0.5 M sodium phosphate, pH 8. The 0.5 M sodium phosphate stock was added to the cis or trans sides of the bilayer to give a final concentration of 10 mM phosphate. The P i -binding experiments were performed with fresh aliquots of (α7) 2 that had been stored at −80 °C, and not thawed more than once. Preparation of liposomes Lipids (25 mg in each case: DPhPC, POPC, POPG and egg-PC, Avanti Polar Lipids) were dissolved in chloroform (1 ml). The stocks of POPC and POPG were mixed to give a molar ratio of POPC:POPG of 9:1. The lipid solutions were dried under a stream of nitrogen, and then kept under high vacuum in a desiccator for 3–4 h. The dried lipids were suspended in rehydration buffer (1 ml of 1 M KCl, 25 mM Tris HCl and 50 μM EDTA, pH 8), and extruded through two 0.1 μm polycarbonate membranes to obtain unilamellar liposomes. For electrical recordings, liposomes (50 or 100 μl) were added to 1 ml recording buffer in the cis compartment. Electron microscopy and image processing To obtain images of (α7) 2 inserted into liposomes, (α7) 2 (50 μg ml −1 ) was mixed with POPC, egg-PC or 10 mol% POPG:POPC liposomes at lipid to protein ratios of 100:1 or 20:1 (w/w), respectively. After incubation for 15–60 min, (α7) 2 was applied to freshly glow-discharged continuous-carbon grids and left to adsorb for 1 min. After blotting, either 2% (w/v) uranyl acetate or NanoVan (Nanoprobes, Inc., USA) was used as a negative stain and applied to the grid for ~15 s. Grids were imaged at either 120 kV (NanoVan) or 80 kV (uranyl acetate), with a Tecnai T12 TEM fitted with a tungsten filament and a BioTWIN lens. Micrographs were recorded on an Eagle 4 k × 4 k charge-coupled device camera with a final pixel size of 1.675 Å per pixel at a nominal magnification of × 52 k. All image processing was performed using EMAN2 [39] . A total of 2,748 particles were selected semiautomatically by using e2boxer and binned by 2. Contrast transfer function parameters were determined using e2ctf, followed by phase flipping and high-pass filtering. Reference-free class averages were generated assuming no symmetry, using e2refine2d. How to cite this article: Mantri, S. et al . An engineered dimeric protein pore that spans adjacent lipid bilayers. Nat. Commun. 4:1725 doi:10.1038/ncomms2726 (2013).